Live cell imaging reveals 3′-UTR dependent mRNA sorting to synapses 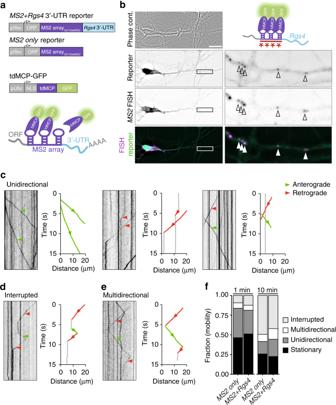Fig. 1 Reporter mRNAs display directed dendritic transport in hippocampal neurons.aScheme of bothMS2 onlyandMS2+Rgs4reporter constructs and tdMCP-GFP expression cassettes (upper) and the MS2 system (lower). pRSV Rous sarcoma virus promoter, pUBC Ubiquitin C promoter, ORF open reading frame, NLS nuclear localization signal, tdMCP tandem MS2 coat protein, UTR untranslated region.bPhase contrast, GFP fluorescence (reporter), MS2 single molecule FISH and overlay in a rat hippocampal neuron expressing both tdMCP-GFP andMS2+Rgs4MS2 reporter mRNA (scheme). Arrowheads indicate overlapping tdMCP-GFP bound MS2 reporter mRNA and MS2 smFISH. Fluorescent images were deconvolved to assess overlap (for unprocessed images see Supplementary Fig.1e). Scale bar 20 µm. Boxed region is magnified in right panels. Representative kymographs (left) and extracted tracks (right) illustrating differences in unidirectionalMS2+Rgs43′-UTR mRNA granule transport speed, displacement and directionality (c), as well as interrupted (d) and multidirectional transport (e). Anterograde and retrograde transport are indicated in green or red arrowheads and lines, respectively.fQuantification of relative transport dynamics ofMS2 onlyandMS2+Rgs43′-UTR reporter mRNAs in 1 and 10-min time-series acquisitions, respectively mRNA transport restricts translation to specific subcellular locations, which is the basis for many cellular functions. However, the precise process of mRNA sorting to synapses in neurons remains elusive. Here we use Rgs4 mRNA to investigate 3′-UTR-dependent transport by MS2 live-cell imaging. The majority of observed RNA granules display 3′-UTR independent bidirectional transport in dendrites. Importantly, the Rgs4 3′-UTR causes an anterograde transport bias, which requires the Staufen2 protein. Moreover, the 3′-UTR mediates dynamic, sustained mRNA recruitment to synapses. Visualization at high temporal resolution enables us to show mRNA patrolling dendrites, allowing transient interaction with multiple synapses, in agreement with the sushi-belt model. Modulation of neuronal activity by either chemical silencing or local glutamate uncaging regulates both the 3′-UTR-dependent transport bias and synaptic recruitment. This dynamic and reversible mRNA recruitment to active synapses would allow translation and synaptic remodeling in a spatially and temporally adaptive manner. Messenger RNAs (mRNAs) display a variety of subcellular localization patterns in a plethora of model systems [1] , [2] , [3] , including the dendritic compartment of the hippocampus [4] . Several distinct mechanisms have been proposed to explain how the sorting of specific mRNAs to subcellular locations can be achieved [2] , [3] , [5] , from simple diffusion to the more complex sushi-belt model of dendritic mRNA trafficking [6] . The latter proposes that mRNA granules patrol dendrites in a highly dynamic multidirectional fashion, without being irreversibly anchored at a single specific location. Multiple approaches demonstrated that specific transcripts can be actively transported along cytoskeletal structures [7] , [8] , [9] . Such active and directed transport has been hypothesized to be the driving force that mediates mRNA sorting to specific distal locations in neurons, such as postsynaptic sites or axonal growth cones, where it may become available for local translation [10] , [11] , [12] , [13] , [14] , [15] . This allows the tightly regulated production of the resulting protein, both spatially and temporally. Localization of mRNA and subsequent local translation are particularly important in neurons, where synapses containing a specific proteome can be located at distal dendrites far from the site of transcription. Ultimately, local protein synthesis at synapses is fundamental for learning and the formation of long-term memory [3] , [6] , [16] , [17] . Previous studies investigated the role of neuronal stimulation on these processes and reported the activity-induced unpacking of mRNAs, allowing local translation in dendrites of primary hippocampal neurons [12] , [18] , [19] , [20] . In addition, glutamate uncaging induces ß-actin mRNA recruitment in dendrites, where it is eventually translated and the newly produced actin participates in dendritic spine remodeling [13] . However, we are only beginning to understand how mRNA is sorted to synapses. 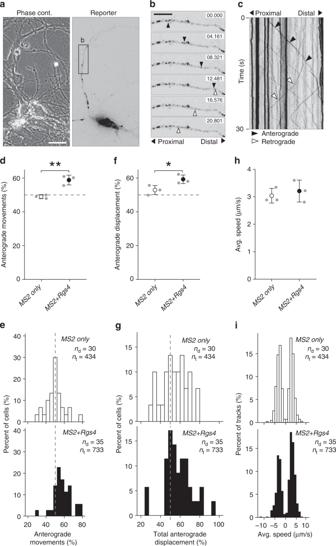Fig. 2 Rgs43′-UTR mediates an anterograde transport bias.aRepresentative phase contrast and GFP fluorescence of hippocampal neuronal culture cotransfected with theMS2+Rgs43′-UTR reporter and tdMCP-GFP constructs. Scale bar 20 µm. Asterisk denotes GFP positive cell.bTime series of the dendritic boxed region ina. Representative anterograde (black arrowheads) and retrograde (white arrowheads) moving mRNA granules are indicated. Scale bars 10 µm.cKymograph of the dendritic region inb. Arrowheads indicate mRNA granules signified inb. Dot plots (d,f,h) and histograms (e,g,i) displaying percentage of anterograde moving granules (d,e), percentage of total anterograde displacement (f,g) and average speed (h,i) forMS2 onlyorMS2+Rgs43′-UTR reporter mRNAs, detected by tdMCP-GFP. In (i), positive values indicate anterograde and negative values indicate retrograde transport. Data represent mean ± standard deviation of three independent experiments (individual experiments shown as gray dots). Asterisks representp-values obtained by Student’sttest (*p< 0.05, **p< 0.01). Data were obtained from 40-µm dendritic segments at a minimal distance of 20 µm from the cell body. At least 10 dendrites/condition/experiment were analyzed. Total number of dendrites (nd) and tracks (nt) analyzed per condition are indicated. Only displacements ≥1.5 µm were considered for analysis Sorting signals, usually within the 3′-untranslated region (3′-UTR) of mRNA, play a crucial role in mRNA localization [2] , [21] , [22] , [23] . Such signals are able to interact with specific RNA binding proteins (RBPs), such as ZBP1, FMRP, or Staufen2 (Stau2), to form neuronal RNA granules [15] , [24] , [25] . Thereby, Stau2 and ZBP1 regulate the dendritic localization of Calm3 and ß-actin mRNA, respectively [26] , [27] . Through these processes RBPs significantly contribute to synaptic function [15] , [28] , [29] . The negative regulator of G protein signaling 4 ( Rgs4 ) mRNA is a physiological target mRNA of Stau2 previously identified in the brain [30] . It encodes a GTPase activating protein of the G protein-coupled receptor (GPCR) pathway, and therefore modulates receptor mediated neuronal signaling at the synapse [31] , [32] , [33] . Fluorescent in situ hybridization (FISH) has shown that Rgs4 mRNA is present in cytosolic RNA granules localized in distal dendrites. Further analysis confirmed the presence of Rgs4 mRNA in Stau2 granules [30] . As the long Rgs4 3′-UTR contains in vivo cross-linking sites for Stau2 [27] , it might provide key binding sites for a direct interaction with Stau2. Silencing of Stau2 induces a reduction of endogenous Rgs4 mRNA both in vitro and in vivo, suggesting an involvement of Stau2 in the regulation of Rgs4 mRNA levels [30] , [34] . To evaluate the role of the 3′-UTR in mediating proper subcellular sorting in mature neurons, we use Rgs4 as a model, and generate an mRNA reporter combining the Rgs4 3′-UTR with an improved MS2 RNA live-cell imaging system [35] , [36] . This reporter system allows us to perform long-term mRNA tracking in dendrites, to (i) unravel the underlying mRNA transport dynamics mediated by a specific 3′-UTR and investigate (ii) neuronal activity and (iii) Stau2 dependency. Together, our results support a model of active, directed mRNA trafficking in a sushi-belt like fashion, promoting synaptic recruitment of mRNA, which would lead to activated translation. This in turn may trigger synaptic remodeling, which ultimately impacts neuronal function. MS2 Rgs4 3′-UTR reporter mRNA localizes to distal dendrites To test whether the 3′-UTR of Rgs4 is sufficient to mediate dendritic localization and to unravel the underlying dynamics of subcellular mRNA sorting, we employed the MS2 system [35] in cultured rat hippocampal neurons. This system makes use of the high affinity and specificity interaction between the MS2 coat protein (MCP) and the MS2 RNA stem-loop structure. We designed mRNA reporters containing the LacZ ORF, followed by a stop codon, an array of either 32 or 128 MS2 stem-loops [36] and the Rgs4 3′-UTR (Fig. 1a ). A second MS2 reporter mRNA lacking the Rgs4 3′-UTR was generated (termed ‘ MS2 only ’ throughout). These reporter mRNAs allowed us to assess the specific contribution of the Rgs4 3′-UTR to dendritic mRNA transport. To visualize the reporter mRNAs in living cells, we cotransfected each reporter plasmid with an expression vector encoding a C-terminally green fluorescent protein (GFP)-tagged tandem MCP (tdMCP-GFP) [37] . A nuclear localization signal (NLS) was included to sequester excess tdMCP-GFP into the nucleus [9] , [35] , [37] , [38] , [39] (Fig. 1a ; Supplementary Fig. 1a ). Expression levels of MS2 only and MS2+Rgs4 reporter mRNAs, tested by RT-qPCR, were comparable (Supplementary Fig. 1b ). Single molecule FISH (smFISH) [40] , targeting the MS2 repeats, demonstrated that the MS2+Rgs4 3′-UTR reporter mRNA localized to dendrites (Supplementary Fig. 1c ), resembling endogenous Rgs4 mRNA [30] . Control reporter mRNAs with no known function in dendrites, i.e. MS2 only or MS2+histone-3.3 3′-UTR, displayed dendritic localization (Supplementary Fig. 1d ). This suggests that dendritic localization is not exclusively dependent on the 3′-UTR, but that other sequences or different expression levels might contribute as well. To further validate the MS2-MCP system in neurons, we cotransfected both the MS2+Rgs4 3′-UTR MS2 reporter and tdMCP-GFP plasmids. GFP fluorescence was clustered in discrete cytoplasmic granules that colocalized with MS2 smFISH signal (Fig. 1b , Supplementary Fig. 1e ), confirming that we reliably detected reporter mRNAs, allowing the visualization of intracellular mRNA transport in living cells. Next, we inquired how specific subcellular sorting within dendrites might be achieved. Fig. 1 Reporter mRNAs display directed dendritic transport in hippocampal neurons. a Scheme of both MS2 only and MS2+Rgs4 reporter constructs and tdMCP-GFP expression cassettes (upper) and the MS2 system (lower). pRSV Rous sarcoma virus promoter, pUBC Ubiquitin C promoter, ORF open reading frame, NLS nuclear localization signal, tdMCP tandem MS2 coat protein, UTR untranslated region. b Phase contrast, GFP fluorescence (reporter), MS2 single molecule FISH and overlay in a rat hippocampal neuron expressing both tdMCP-GFP and MS2+Rgs4 MS2 reporter mRNA (scheme). Arrowheads indicate overlapping tdMCP-GFP bound MS2 reporter mRNA and MS2 smFISH. Fluorescent images were deconvolved to assess overlap (for unprocessed images see Supplementary Fig. 1e ). Scale bar 20 µm. Boxed region is magnified in right panels. Representative kymographs (left) and extracted tracks (right) illustrating differences in unidirectional MS2+Rgs4 3′-UTR mRNA granule transport speed, displacement and directionality ( c ), as well as interrupted ( d ) and multidirectional transport ( e ). Anterograde and retrograde transport are indicated in green or red arrowheads and lines, respectively. f Quantification of relative transport dynamics of MS2 only and MS2+Rgs4 3′-UTR reporter mRNAs in 1 and 10-min time-series acquisitions, respectively Full size image Rgs4 3′-UTR-dependent anterograde transport bias in dendrites To investigate dynamics underlying mRNA transport, time-lapse imaging of single neurons expressing the MS2 system was performed for 1 min at 15.3 fps (frames per second) with a spinning disk microscope. To analyze the characteristics of single trafficking RNA granules, we generated kymographs of dendritic regions at a minimal distance of 20 µm from the soma and traced single trajectories (Figs. 1 c–e; 2a–c ; Supplementary Movies 1 – 8 ). This revealed diverse RNA transport patterns, independent of a 3′-UTR. We observed mobile mRNA granules with differences in transport speed, displacement length and directionality (Fig. 1c , Supplementary Movies 1 – 3 ). Furthermore, two additional distinct types of mRNA granule mobility were detected. We found that mRNA granules may interrupt their movement before reinitiating transport (Fig. 1d , Supplementary Movie 4 , interrupted) or may display multiple changes in direction without interrupting transport (Fig. 1e , Supplementary Movies 5 and 6 , multidirectional). In addition, we observed mRNA granules that reversed direction at dendritic branch points to move between different segments (Supplementary Movie 7 ). These transport behaviors support the sushi-belt model of dendritic mRNA trafficking, which proposes that mRNA granules patrol dendrites in a highly dynamic multidirectional fashion, without being irreversibly anchored at a single specific location [6] . We quantified the frequencies of these transport behaviors and found that half of the mRNA granules remained stationary during the 1 min acquisition period. In contrast, the mobile fraction of granules traversed the dendrites in a highly dynamic way, including unidirectional, interrupted, and multidirectional movements, independent of the 3′-UTR (Fig. 1f ). Increasing the acquisition time to 10 min reduced the fraction of stationary and unidirectional granules in favor of interrupted and multidirectional movements, demonstrating that a large fraction of RNA granules indeed undergo transport in a sushi-belt like fashion. The fraction of the stationary population is consistent with previously published data for the ß-actin mRNA as well as for Staufen1 granules in the time frames analyzed [13] , [41] . Statistical analysis by the Chi-squared test could not establish any difference in the frequency of these events between MS2 only or MS2+Rgs4 3′-UTR reporter mRNAs, suggesting that the 3′-UTR of the transcript does not regulate the types of motility exhibited by the reporters. As both MS2+Rgs4 and MS2 only reporter mRNAs were found to be localized in dendrites, we decided to investigate the underlying regulation of dendritic mRNA sorting, which ultimately fine-tunes trafficking to achieve a specific localization upon demand. We examined multiple parameters of 3′-UTR-dependent mRNA granule transport, including speed, displacement and directionality in dendrites (Fig. 2 ; Supplementary Fig. 2 ; Supplementary Movie 8 ). When exploring transport directionality, the MS2 only mRNA displayed an equal number of mRNA granules moving in the anterograde (48.9 ± 1.2%) or retrograde direction (Fig. 2d, e ). Interestingly, the MS2+Rgs4 3′-UTR mRNA mediated a significant anterograde transport bias, with 58.8 ± 2.9% of mRNA granules moving toward more distal dendritic regions (Fig. 2d, e ; p = 0.0056). Moreover, when the percentage of total anterograde travel distance of all mRNA granules was investigated, we observed a similar transport bias for the MS2+Rgs4 3′-UTR (59.1 ± 2.5%) compared to the MS2 only (52.8 ± 2.6%) mRNA reporter (Fig. 2f, g ; p = 0.0399). Directional transport has previously been observed for other mRNAs, such as ß-actin , Arc , and CaMKIIα , in hippocampal neurons or oskar in the Drosophila oocyte, with a preferential transport direction toward the distal or the posterior part of the cell, respectively [9] , [38] , [39] , [42] . In contrast, we observed no differences in either average transport speed or in average displacement length of single events, indicating that the Rgs4 3′-UTR did not affect these parameters of mRNA transport (Fig. 2h, i ; Supplementary Fig. 2a, b ). The distribution of single data points showed that most RNA granules underwent short displacement events and only few particles traveled long distances at a time, often longer than the 40 µm analyzed (Supplementary Fig. 2b ). To exclude that the NLS fused to the tdMCP protein might potentially affect transport as previously reported [43] , we generated a tdMCP lacking the NLS and repeated the previous experiment. Although this yielded a higher fluorescent background, we still observed an anterograde transport bias mediated by the Rgs4 3′-UTR (Supplementary Fig. 2c, d ), showing that the NLS did not affect trafficking in our hands. Fig. 2 Rgs4 3′-UTR mediates an anterograde transport bias. a Representative phase contrast and GFP fluorescence of hippocampal neuronal culture cotransfected with the MS2+Rgs4 3′-UTR reporter and tdMCP-GFP constructs. Scale bar 20 µm. Asterisk denotes GFP positive cell. b Time series of the dendritic boxed region in a . Representative anterograde (black arrowheads) and retrograde (white arrowheads) moving mRNA granules are indicated. Scale bars 10 µm. c Kymograph of the dendritic region in b . Arrowheads indicate mRNA granules signified in b . Dot plots ( d , f , h ) and histograms ( e , g , i ) displaying percentage of anterograde moving granules ( d , e ), percentage of total anterograde displacement ( f , g ) and average speed ( h , i ) for MS2 only or MS2+Rgs4 3′-UTR reporter mRNAs, detected by tdMCP-GFP. In ( i ), positive values indicate anterograde and negative values indicate retrograde transport. Data represent mean ± standard deviation of three independent experiments (individual experiments shown as gray dots). Asterisks represent p -values obtained by Student’s t test (* p < 0.05, ** p < 0.01). Data were obtained from 40-µm dendritic segments at a minimal distance of 20 µm from the cell body. At least 10 dendrites/condition/experiment were analyzed. Total number of dendrites ( n d ) and tracks ( n t ) analyzed per condition are indicated. Only displacements ≥1.5 µm were considered for analysis Full size image In conclusion, our live-cell imaging data suggest that the Rgs4 3′-UTR was responsible for the observed anterograde transport bias, affecting both anterograde moving mRNA granule number and anterograde travel distance in dendrites. Importantly, the results establish the 3′-UTR as a key determinant, as the bias was not observed in the absence of the Rgs4 3′-UTR. Neuronal inhibition abolishes the Rgs4 3′-UTR transport bias Next, we asked whether neuronal activity might regulate dendritic mRNA transport. As mature neurons display endogenous neuronal activity in culture, we chemically silenced activity by simultaneously inhibiting AMPA receptors, NMDA receptors, and voltage-gated sodium channels via bath application of CNQX, AP5, and TTX [27] . Neurons transfected with either MS2 only or MS2+Rgs4 3′-UTR reporters were left untreated or preincubated for 1 h with either vehicle or CNQX/AP5/TTX, and then imaged during continuous treatment (Fig. 3a ). No differences in speed, displacement, or transport directionality were observed for the MS2 only mRNA reporter, independent of treatment (Fig. 3b, c , Supplementary Fig. 3a, b, g, h ; displacement (µm): untreated 5.6 ± 6.7, DMSO 5.5 ± 6.9, silenced 6.2 ± 7.1). However, when neuronal activity was inhibited the anterograde transport bias mediated by the MS2+Rgs4 3′-UTR was completely abolished (46.7 ± 2.3%), compared to vehicle treated (55.1 ± 2.9%, p = 0.00431) or untreated neurons (56.3 ± 2.3%, p = 0.00187) (Fig. 3d, e ; F 2,9 = 0.00136). Moreover, the inhibition of neuronal activity alleviated the anterograde bias observed in respect to total travel distance (50.2 ± 2.5%), compared to vehicle treated samples (56.0 ± 3.0%, p = 0.02884) (Supplementary Fig. 3c, d ). Importantly, these effects were not due to neuronal toxicity, as 1 h wash-off of chemical inhibition induced recovery of the transport bias ( F 2,9 = 0.00093, p = 0.01456 for silenced vs wash-off, p = 0.00074 for silenced vs untreated, Fig. 3f, g ). Anterograde displacement of MS2+Rgs4 3′-UTR mRNA granules partially recovered after 1 h wash-off ( F 2,9 = 0.021, p = 0.424 for silenced vs wash-off, p = 0.017 for silenced vs untreated, Supplementary Fig. 3e, f ). Moreover, fractions of mRNA granule mobility, categorized as stationary, unidirectional, interrupted, and multidirectional, remained unaffected by inhibition of neuronal activity (Supplementary Fig. 3i, j ). Evaluation of mRNA expression levels in cortical neurons by RT-qPCR and independent quantification of dendritic mRNA granules in single hippocampal neurons showed that neuronal inhibition did not affect either the amount of reporter mRNAs or mRNA granules analyzed (Supplementary Fig. 4a, b ). Together, these data demonstrate that the transport bias of the reporter mRNAs not only depended on the Rgs4 3′-UTR, but on neuronal activity as well. Importantly, the movement of the MS2 only mRNA reporter remained unaffected by synaptic inhibition, suggesting that neuronal silencing did not reduce the mRNA transport bias in general, but that the effect was indeed dependent on the Rgs4 3′-UTR. Fig. 3 Inhibition of neuronal activity abolishes Rgs4 3′-UTR-dependent transport bias. a Scheme of experimental outline. Dot plots ( b , d , f ) and histograms ( c , e , g ) displaying percentage of anterograde moving MS2 only ( b , c ) or MS2+Rgs4 3′-UTR ( d – g ) reporter mRNA granules in rat hippocampal neurons, untreated, vehicle treated (DMSO) or silenced (100 µM CNQX, 50 µM AP5, 1 µM TTX) and after 1-h recovery. Data represent mean ± standard deviation of 3–4 independent experiments (individual experiments shown as gray dots). Asterisks represent p -values assessed by Tukey’s test post-hoc to one-way ANOVA analysis (* p < 0.05, ** p < 0.01, *** p < 0.001). Data were obtained from 40-µm dendritic segments at a minimal distance of 20 µm from the cell body. At least 10 dendrites/condition/experiment were analyzed. Total number of dendrites ( n d ) and tracks ( n t ) analyzed per condition are indicated. Only displacements ≥1.5 µm were considered for analysis Full size image Rgs4 3′-UTR-dependent mRNA sorting to synapses As inhibition of neuronal activity abolished the Rgs4 3′-UTR-dependent anterograde transport bias in distal dendrites, we next investigated whether mRNA was recruited to dendritic synapses. To visualize endogenous excitatory synapses in dendrites, we generated a fluorescent synaptic marker by tagging the postsynaptic density protein 95 kD (PSD-95) with tagRFPt (PSD-95-RFP). Mature neurons were cotransfected with PSD-95-RFP, tdMCP-GFP and either the MS2 only or MS2+Rgs4 3′-UTR mRNA reporters. To analyze whether synapses might affect mRNA granule transport, we coimaged both mRNA reporters and the synaptic marker by time-lapse dual-color microscopy in single cells for 1 min. We generated kymographs for each separate channel and created dual-color overlays (Fig. 4a ; Supplementary Movies 9 and 10 ). We identified the positions, where mRNA granules were found to either interrupt (termed docking) or reinitiate transport (termed undocking), and measured the distance to the closest PSD-95-RFP positive cluster. Importantly, co-expression of the fluorescent reporters together with either MS2 only or MS2+Rgs4 3′-UTR reporter mRNA did not modify synaptic density (Supplementary Fig. 5a ). Moreover, we found no difference in the ratio of mRNA granules docking or undocking between MS2 only and MS2+Rgs4 3′-UTR reporter mRNAs, respectively (Supplementary Fig. 5b ). While both reporter mRNAs were recruited to synapses, MS2+Rgs4 3′-UTR reporter mRNAs on average docked closer than MS2 only reporter mRNAs (1.11 ± 0.01 µm for MS2 only vs 0.67 ± 0.02 µm for MS2+Rgs4 3′-UTR; p = 4.25E −6 , Fig. 4b, c ). Similar results were obtained for mRNA granules undocking after a previous stationary phase (Supplementary Fig. 5c, d ). Together, these results suggest a dynamic sorting process as the Rgs4 3′-UTR mediated mRNA recruitment and eventual release close to synapses. Fig. 4 Rgs4 3′-UTR mediates mRNA recruitment to synapses dependent on neuronal activity. a Representative dual-color kymograph showing MS2+Rgs4 3′-UTR reporter mRNA (green) and PSD-95-tagRFPt (magenta) from a dendrite of a rat hippocampal neuron. First and last frames are shown at top and bottom. Scale bar 5 µm. Extracted track (right) of an mRNA granule docking at a PSD-95 positive area indicated by arrowheads. Distance of MS2 only or MS2+Rgs4 3′-UTR reporter mRNA docking events to closest PSD-95 positive cluster in neurons displayed as dot plot ( b ) and density plot ( c ). d Distribution of MS2 only or MS2+Rgs4 reporter mRNA-positive (estimated RNA number ≥1 at t = 0 s) and -negative (RNA = 0 at t = 0 s) PSD-95-tagRFPt clusters in soma and dendrites. P-values of Chi [2] tests against control are indicated. e Integrated frequency of reporter docking and undocking events at dendritic synapses. Number of observations and population means are indicated. f Average net change of MS2 only or MS2+Rgs4 mRNA content at mRNA reporter-positive or -negative synapses per min, calculated from estimated reporter molecules docking or undocking at synapses per event. Numbers indicate mean value of net RNA level change. Error bars represent 95% confidence intervals. ** indicates significant ( α = 0.01) difference compared to zero (null hypothesis, two sided one-sample t -test). Distance of MS2+Rgs4 3′-UTR reporter mRNA docking events to closest PSD-95 positive cluster under untreated, vehicle treated (DMSO) or silenced (100 µM CNQX, 50 µM AP5, 1 µM TTX) conditions displayed as dot plot ( g ) and density plot ( h ). Data represent mean ± standard deviation of three independent experiments (individual experiments shown as gray dots; b , g ). Dashed lines represent mean values of single data points ( c , h ). Asterisks represent p -values obtained by Student’s t test ( b ), Mann Whitney U test ( e ) or Tukey’s test post-hoc to one-way ANOVA analysis ( g ) (** p < 0.01, *** p < 0.001). Data were obtained from 40-µm dendritic segments at a minimal distance of 20 µm from the cell body. At least 10 dendrites/condition/experiment ( a – c , g , h ) or 12 neurons/condition ( d – f ) from 3 independent biological replicates were analyzed. Total number of dendrites ( n d ), events ( n e ) and synapses ( n ) analyzed per condition are indicated Full size image To further investigate how MS2 only and MS2+Rgs4 3′-UTR RNA reporters behave at the synapse, we acquired longer dual-color videos (3.5 min, at ~4.7 fps) of neurons cotransfected with either MS2 only or the MS2+Rgs4 , tdMCP-GFP and the synaptic marker PSD-95-RFP. We tracked PSD-95-RFP positive clusters over time and measured the GFP fluorescence of reporter mRNAs in equivalent areas. This allowed us to specifically analyze dynamic changes in GFP fluorescence intensity caused by docking or undocking reporter mRNAs at single synapses (see “Methods” for details). During the time analyzed, we observed at least one docking or undocking event of either MS2 only or MS2+Rgs4 reporter mRNAs at ~34% vs ~21% of dendritic synapses, respectively (Supplementary Fig. 5e ). This represents a ~30% significant reduction in the frequency of these events for the MS2+Rgs4 3′-UTR reporter mRNA ( p < 0.0001; Supplementary Figs. 5f and 6d ). We found that the number of these events showed a moderate correlation ( R ~ 0.5) with the estimated mRNA copy number within PSD-95-RFP positive synapses (Supplementary Fig. 5g ). This suggests that the number of docking/undocking events is related with the total number of mRNA particles at synapses. Analysis of the postsynaptic sites revealed that mRNA-positive synapses were both larger and brighter in their mean PSD-95 signal intensity than mRNA negative synapses ( p < 0.0001; Supplementary Fig. 5h ). We found that the fraction of MS2+Rgs4 3′-UTR positive synapses in dendrites was significantly lower than that of MS2 only (57.1% vs 73.9%; p < 0.0001; Fig. 4d ). However, when we focused on mRNA reporter-positive synapses, we found a significant but nonsubstantial difference between the frequency of total docking/undocking events of MS2 only and MS2+Rgs4 3′-UTR reporter mRNAs at synapses ( p = 0.002; Fig. 4e ). Subsequently, we analyzed the net directionality of reporter mRNA docking or undocking events separately at postsynaptic densities. We found that the frequency of docking events was significantly higher for the MS2+Rgs4 , compared to the MS2 only reporter (~0.9 min −1 for MS2+Rgs4 vs 0.79 min −1 for MS2 only , p = 0.005), whereas there was no substantial difference in the frequency of undocking events (~0.99 min −1 for MS2+Rgs4 vs 0.97 min −1 for MS2 only ). In agreement with these results, we found a net influx ( p = 0.009, α = 0.01) of MS2+Rgs4 into mRNA-positive synapses, in contrast to the MS2 only reporter mRNA (Fig. 4f , Supplementary Fig. 4i ), which was not significantly different from zero ( p = 0.043, α = 0.01). In general, synapses contained mRNA at the beginning and during the experiment regardless of their location and reporter mRNA (Supplementary Fig. 6a–d ). In summary, these data demonstrate that the MS2+Rgs4 3′-UTR-mediated docking in closer proximity to synapses, compared to the MS2 only 3′-UTR. Furthermore, although the MS2+Rgs4 reporter interacted with fewer synapses, it displayed a net increase at synapses, while the MS2 only reporter did not. These findings suggest that dendritically localized MS2+Rgs4 mRNA was associated with a specific subset of synapses. Neuronal activity recruits Rgs4 3′-UTR mRNA to synapses Next, we investigated whether inhibition of neuronal activity affected recruitment of Rgs4 3′-UTR mRNA to synapses in addition to its effect on transport directionality. Therefore, we chemically inhibited neuronal activity in mature rat hippocampal neurons transiently cotransfected with either the MS2 only or the MS2+Rgs4 3′-UTR mRNA, tdMCP-GFP and the synaptic marker PSD-95-RFP. Neither synaptic density nor the ratio of docking to undocking events was altered when silenced cells were compared with vehicle or untreated controls (Supplementary Fig. 7a, b ). In addition, MS2 only mRNA granules did not exhibit any significant change in their distance to PSD-95-RFP synapses upon inhibition of neuronal activity when compared to vehicle or untreated cells (Supplementary Fig. 7c, d ). However, the inhibition of neuronal activity increased the docking/undocking distance of MS2+Rgs4 mRNA close to synapses, to values comparable to MS2 only mRNA ( F 2,6 = 0.001, p = 0.004 for silencing vs vehicle, p = 0.001 for silencing vs untreated, Fig. 4g, h ; F 2,6 = 0.001, p = 0.003 for silencing vs vehicle, p = 0.00162 for silencing vs untreated, Supplementary Fig. 7e, f ). Next, we performed local two-photon glutamate uncaging at individual dendritic spines to evaluate whether the stimulation of single spines would be sufficient to recruit mRNA granules. Either the MS2 only or the MS2+Rgs4 reporter mRNAs were cotransfected with tdMCP-GFP and tandem Tomato (tdTomato). Upon glutamate uncaging adjacent to individual spines, we observed an increase in spine size by the volume marker (tdTomato) (Supplementary Fig. 8a ). The mRNA granule number before and after uncaging was quantified within a 5 µm radius along dendrites centered at the stimulated spine. We observed an average increase of ~3 RNA granules for the MS2+Rgs4 reporter mRNA, while there was no increase of MS2 only reporter granules (Fig. 5a, b , Supplementary Fig. 8b , Supplementary Movie 11 ). Together, these data demonstrate that neuronal activity is not only necessary to mediate the Rgs4 3′-UTR-dependent mRNA transport bias, but is also required to recruit its mRNA to activated synapses. Furthermore, we provide further experimental evidence that it is the Rgs4 3′-UTR that has a direct influence on activity-dependent mRNA docking/undocking, as the MS2 only reporter mRNA remained unaffected by neuronal inhibition or local stimulation of dendritic spines. Fig. 5 Local glutamate uncaging at spines triggers Rgs4 3′-UTR-dependent mRNA recruitment. a Representative GFP fluorescence of a hippocampal neuron cotransfected with the MS2+Rgs4 3′-UTR reporter and tdMCP-GFP constructs before (left panel) and after (middle, right panels) local glutamate uncaging. Black arrowhead denotes the uncaging spot at dendritic spine. White arrowheads indicate GFP positive MS2+Rgs4 reporter mRNA granules. Scale bar 2 µm. b Dot plot displaying the change in RNA granule number 40–45 min after uncaging compared to before uncaging within 5 µm of the stimulated spine. Data represent mean ± standard deviation (individual neurons shown as gray dots). Asterisks represent p -values obtained by Student’s t test (*** p < 0.001). Data were obtained from six dendrites for MS2 only (five neurons of four biological replicates) and five dendrites for MS2+Rgs4 reporter mRNAs (five neurons of five biological replicates), respectively Full size image Stau2 regulates dendritic transport via the Rgs4 3′-UTR Finally, we investigated whether the RBP Stau2, which is known to bind Rgs4 mRNA [27] , [30] , was required for the transport of MS2+Rgs4 granules. To examine whether mRNA is cotransported with Stau2, we cotransfected the MS2+Rgs4 reporter with tdMCP-GFP and tagRFPt-tagged Stau2 (RFP-Stau2). We observed multiple instances, where the MS2+Rgs4 reporter mRNA granules were cotransported with Stau2 (Fig. 6a , Supplementary Movies 12 - 13 ). Moreover, overexpression of Stau2 resulted in an increase of dendritic MS2+Rgs4 reporter density, while the MS2 only mRNA was unaffected (Supplementary Fig. 9a ). In addition, we performed an experiment involving MS2 RNA-mediated tethering of Stau2 to the MS2 only reporter mRNA. When we cotransfected both tdMCP-Stau2 and tdMCP-GFP together with the MS2 only reporter, we observed that the tethering of Stau2 tended to recruit the control mRNA closer to the synaptic marker vesicular glutamate transporter 1 (VGLUT1) (Supplementary Fig. 9b ). Together, our data suggest that Stau2 might indeed regulate Rgs4 3′-UTR-dependent recruitment to synapses. However, additional work is clearly necessary to substantiate these findings in the future. Fig. 6 Stau2 regulates Rgs4 3′-UTR-dependent transport. a Representative dual-color kymograph showing MS2+Rgs4 3′-UTR reporter mRNA (green) and tagRFPt-tagged Stau2 (magenta) from a dendrite of a rat hippocampal neuron. First and last frames are shown at top and bottom. Arrowheads indicate an MS2+Rgs4 reporter and Stau2 positive RNA granule undergoing cotransport. Scale bar 5 µm. Dot plots ( b , d ) and histograms ( c , e ) displaying percentage of anterograde moving MS2 only or MS2+Rgs4 3′-UTR reporter mRNA granules in shNTC and shStau2 transduced hippocampal neurons. NTC non-targeting control. Data represent mean ± standard deviation of three independent experiments (individual experiments shown as gray dots). Asterisks represent p -values obtained by Student’s t test (* p < 0.05). Data were obtained from 40-µm dendritic segments at a minimal distance of 20 µm from the cell body. Total number of dendrites ( n d ) and tracks ( n t ) analyzed per condition are indicated. Only displacements ≥1.5 µm were considered for analysis Full size image To further investigate the involvement of Stau2 in dendritic mRNA transport, we transduced neurons with lentiviral particles expressing either a short hairpin nontargeting control (shNTC) or a short hairpin specific for Stau2 (shStau2-2) [28] 4 days prior to cotransfection with tdMCP-GFP and MS2 only or MS2+Rgs4 3′-UTR reporter mRNAs. Time-lapse imaging revealed that the MS2 only reporter mRNA remained unaffected by Stau2 knockdown (Fig. 6b, c , Supplementary Fig. 9c, d ). In contrast, Stau2 knockdown abolished the anterograde transport bias of MS2+Rgs4 3′-UTR mRNA granules in distal dendrites ( p = 0.012, Fig. 6d, e ). Total anterograde displacement remained unaffected for MS2 only mRNA, but showed a nonsignificant reduction for the MS2+Rgs4 3′-UTR reporter in Stau2 deficient neurons (Supplementary Fig. 9e, f ). Different types of MS2+Rgs4 3′-UTR mRNA granule mobility, categorized as stationary, unidirectional, interrupted and multidirectional, as well as speed and displacement length were unaffected by Stau2 knockdown (Supplementary Fig. 9g ; speed (µm s −1 ): shNTC 3.2 ± 1.3, shStau2 2.9 ± 1.2; displacement (µm): shNTC 6.9 ± 7.5, shStau2 6.5 ± 6.5). The reduction of Stau2 expression was verified in the imaged samples by immunostaining (Supplementary Fig. 10a ). Moreover, quantification by RT-qPCR revealed that Stau2 knockdown did not affect the expression levels of reporter mRNAs (Supplementary Fig. 10b ). In conclusion, these data provide direct experimental evidence that Stau2, which is cotransported together with Rgs4 reporter mRNA in distinct RNA granules, is responsible for the observed 3′-UTR-dependent transport bias. Here, we show that mRNAs travel along dendrites in a dynamic and multidirectional fashion, a process that does not exclusively require a specific 3′-UTR. The presence of the Rgs4 3′-UTR, however, conveyed key properties to the reporter mRNA, which fine-tune transport as (i) it introduced a transport bias directed toward distal dendrites, and (ii) regulated the spatio-temporal association with synapses. This was dependent on neuronal activity and the RBP Stau2. Together, our data not only provide experimental support for the sushi-belt model of dendritic mRNA transport [6] , in which mRNAs dynamically patrol synapses, but also allow us to advance this model by the introduction of a regulated transport bias. This sheds mechanistic insight into global RNA sorting processes, including recruitment of RNAs by individual stimulated synapses. Here, we present evidence that mRNA granules traverse distal dendrites in a directed manner, independently of the presence of a specific 3′-UTR. All MS2 only , MS2+Rgs4 and MS2+histone-3.3 3′-UTR mRNA reporters formed dendritic mRNA granules, suggesting that additional factors other than 3′-UTR sequences contribute to dendritic localization. For instance, the poly-A-tail or other mRNAs contained in the same granule [3] might be involved. However, independently of the 3′-UTR sequence, a proportion of the observed RNA granules remained stationary, while others showed variability in speed, displacement length, and directionality of transport. In addition to both simple anterograde and retrograde transport, some mRNA granules displayed more complex dynamics. Indeed, some granules interrupted and subsequently reinitiated transport or even switched direction without interruption. This interrupted transport has recently been investigated and computationally modeled, providing a basis for future functional studies [44] . In addition, we show here that longer observation time revealed an increase in interrupted movements and a decrease in unidirectional or stationary phases, demonstrating that a majority of mRNA granules may undergo multiple transport phases in different directions. This observation expands our current understanding of mRNA sorting beyond local recruitment, as it proves experimentally that mRNA granules are not irreversibly anchored, but are dynamic, can be targeted to specific sites upon demand, and be released from them later on. Taken together, we provide experimental evidence that the sushi-belt model accurately describes dendritic mRNA transport in live neurons. However, we do not exclude that other factors/mechanisms might contribute as well. Interestingly, a recent computational study provides evidence that the sushi-belt model can achieve complex spatial distribution of cargo in neurons [45] . A key finding of the current study is that the 3′-UTR of Rgs4 mRNA mediated an anterograde transport bias in dendrites, i.e. preferential transport directionality toward distal regions. In contrast, neither the MS2 only nor the MS2+histone-3.3 reporter mRNAs displayed this bias (Fig. 2d ; MS2+histone-3.3 anterograde movement (%): 51.2 ± 0.3). Previous studies have observed both anterograde and retrograde mRNA transport. However, a directional bias in transport has been reported only in few cases, e.g. for oskar mRNA in the Drosophila oocyte, or for ß-actin and Arc mRNAs in mouse hippocampal neurons [9] , [38] , [42] , [46] . It is worth mentioning that these studies observed a bias of similar magnitude as we report here (~60% toward distal regions), indicating that the dendritic bias of the MS2+Rgs4 3′-UTR reporter is within a physiological range. Interestingly, silencing of neuronal activity abolished the MS2+Rgs4 3′-UTR specific transport bias, while the transport of the MS2 only reporter remained unaffected. Endogenous neuronal signaling in culture restored the bias, demonstrating its physiological pertinence. In contrast to our observations, Arc mRNA transport bias was not affected by neuronal activity [46] . This suggests that anterograde transport is differentially regulated depending on mRNA sequence and that distinct RNA granules may be differently regulated by neuronal activity. Furthermore, we show that knockdown of Stau2 abolished the Rgs4 3′-UTR-dependent anterograde transport bias as well. As the MS2 only reporter mRNA remained unaffected by Stau2 knockdown, the loss of the anterograde transport bias is specific to the Rgs4 3′-UTR and might be caused by the absence of Stau2 in Rgs4 containing mRNA granules. Therefore, we hypothesize that Stau2 might be recruited in conjunction with neuronal activity to modulate dendritic Rgs4 mRNA transport. Similarly, previous research has shown how Staufen and other RBPs are not necessary for general transport, but can facilitate or modulate it [47] , [48] . Along this line, Staufen has been implicated in kinesin-1-dependent posterior localization of oskar mRNA in Drosophila and has been found in a complex with kinesin-1 in Xenopus [47] , [48] . In line with this finding, we observed directed cotransport of MS2+Rgs4 granules together with Stau2 in neurons. Importantly, Stau2 depletion results in both morphological and physiological synaptic phenotypes [28] , [49] . Therefore, it is tempting to speculate that Stau2 might not only regulate the expression of proteins relevant at synapses as previously shown [30] but also the transport and recruitment of their mRNAs. In turn, deregulation of synaptic proteins, resulting in aberrant synaptic remodeling, might render a synapse incapable to properly recruit relevant transcripts. Together, our data give functional insight into the regulation of 3′-UTR-dependent mRNA transport. We show that it is the Rgs4 3′-UTR that facilitates dendritic localization via the anterograde transport bias. Although dendritic sorting might be affected by other factors such as regulated mRNA degradation, this transport bias might enable fast and efficient mRNA recruitment to specific regions such as synapses as needed. Future studies will have to unravel the detailed molecular mechanisms of how Stau2, neuronal activity and 3′-UTR sequences cooperate to mediate this anterograde bias in neurons. Another key observation is that the MS2+Rgs4 3′-UTR facilitated mRNA docking and undocking in closer proximity to synapses compared to MS2 only . Upon silencing of endogenous neuronal activity, the distance of docking/undocking was increased for the MS2+Rgs4 3′-UTR, while the MS2 only reporter remained unaffected. Conversely, local stimulation of individual dendritic spines by glutamate uncaging resulted in increased recruitment of MS2+Rgs4 granules, but not MS2 only mRNAs. Furthermore, the MS2+Rgs4 3′-UTR reporter interacted with fewer synapses and displayed more docking events at dendritic synapses than the MS2 only reporter. This led to a slower turnover of MS2+Rgs4 mRNA content at synapses compared to MS2 only , indicating MS2+Rgs4 is more stably associated and might remain at synapses longer. We propose that the presence of MS2 only mRNA at synapses might represent a state of nonspecific, default localization. These effects, along with the observed differences in the brightness of PSD-95 clusters could reflect differences in either synaptic activity or in the subtype of synapses. As the Rgs4 protein is a negative regulator of synaptic activity, we speculate that its mRNA is transported to a subtype of synapses, where it might be regulated in situ. Here, the mRNA could be unpacked and locally translated by polysomes localized close to PSD-95 clusters [50] , where the newly synthesized Rgs4 protein would modulate GPCR-mediated neuronal signaling. Our findings are in agreement with a study by the Singer lab that showed that endogenous ß-actin mRNA is recruited to glutamate-stimulated dendritic spines, where it is locally translated [13] . Using a similar approach, we now show that glutamate stimulation of individual spines results in 3′-UTR-dependent recruitment of Rgs4 mRNA, as the MS2 only reporter displayed no variation in recruitment. In conclusion, we hypothesize that the observed anterograde transport bias contributes to synaptic recruitment of mRNAs. As both the transport bias and synaptic recruitment are modulated by the 3′-UTR and neuronal activity, anterograde transport might indeed facilitate synaptic recruitment, especially at endogenous mRNA expression levels. Future work will aim to understand how neuronal activity affects the organization of key cytoskeletal components to mediate Rgs4 mRNA recruitment and whether it affects their capture on ribosomes at synapses. We therefore propose a model of Rgs4 trafficking in neuronal Stau2 mRNA granules, in which its 3′-UTR specifically mediates sorting to distal dendrites. In this model, the Rgs4 mRNA patrols the dendrite in a dynamic fashion in accordance with the sushi-belt model [6] . Neuronal activity can result in the docking of this mRNA at specific postsynaptic sites and cause unpacking of the mRNA from transport granules. There, the mRNA may be subjected to local translation, making the encoded Rgs4 protein available in a spatially and temporally restricted manner. After the mRNA has fulfilled its function at the synapse, it may undock and reinitiate transport until it is degraded or recruited for a new round of translation. Such processes are the basis of cellular mechanisms in polarized cells involved in, e.g. dendritic arborization, long-term potentiation, and synaptic plasticity and are indispensable for neuronal development, learning, and memory formation. Neuronal cell culture, transfection and transduction Rat hippocampal neuronal cell cultures [51] were generated as follows: hippocampi of embryonic day 17 (E17) embryos of timed pregnant Sprague-Dawley rats (Charles River Laboratories) were isolated, cells dissociated with 2.5% trypsin and plated on poly- l -lysine coated coverslips or glass bottom dishes (WillCo Wells) and cultured in NMEM+B27 medium (Invitrogen) at 37 °C with 5% CO 2 . In case of cortical cultures, E17 cortices were dissociated, the cell suspension sequentially filtered through 100- and 70-μm filters and then plated at a density of 700 cells/mm 2 . Experiments were performed with cultured neurons between 10 and 16 days in vitro (DIV). Neurons were transiently transfected by calcium phosphate coprecipitation [52] at 10–15 DIV and imaged at 11–16 DIV. For each transfection condition 3–5 μg of DNA was mixed with 6 μl of 2.5 M CaCl 2 , in a final volume of 60 μl. Then, 60 μl of 2× BES buffer (pH = 7.00–7.20) was added to the mixture dropwise and air bubbles were introduced to the solution with the pipette. Each component was added stepwise and slowly. This mixture was added to the neurons and the precipitate was incubated with the cells under atmospheric CO 2 concentration for 1 h at 37 °C. For experiments involving glutamate uncaging, neurons were plated on poly- l -lysine and laminin (Invitrogen) coated 12-mm-diameter glass coverslips, at a density of 600 cells/mm 2 . Cells were transfected at 15–17 DIV by calcium phosphate coprecipitation and imaged the following day. To knockdown Stau2 expression, 10–11 DIV neurons were transduced overnight with lentiviral suspension, transfected with MCP-GFP and MS2 mRNA reporter constructs at 14–15 DIV and imaged at 15–16 DIV or lysed for RNA extraction. All animals were used according to the German Welfare for Experimental Animals (LMU Munich, Regierung von Oberbayern ). Human embryonic kidney 293T (HEK-293; ATCC CRL3216) cells were grown in Dulbecco’s modified Eagle’s medium (DMEM; Invitrogen) supplemented with 10% fetal bovine serum (FBS; Invitrogen), stable 1% l -alanyl- l -glutamine (Biochrom) and 1% sodium pyruvate (Sigma Aldrich), and incubated at 37 °C with 5% CO 2 . One day before transfection, HEK-293 cells were plated in six-well plates at 5 × 10 4 cells/well and transfected with indicated plasmids using calcium phosphate protocol. Plasmids RNA reporter constructs were placed under the control of an RSV promoter, together with LacZ as ORF, a stop codon, and an array of either 32 unique MS2 hairpins or a quadruplication of this array, i.e. 128 MS2 hairpins [36] . The 3′-UTR was either omitted (pRSV-LacZ-MS2) or included (pRSV-LacZ-MS2- Rgs4 3′-UTR or pRSV-LacZ-MS2- H3.3 3′-UTR) prior to the poly-A signal. Sequences of the 3′-UTRs correspond to the positions 728–2919 nt of rat Rgs4 mRNA (NM_017214.1) or 537–1087 nt of rat Histone3.3 mRNA (X73683.1). To generate the pUBC-NLS-ha-tdMCP-GFP plasmid, the nls-HA-tdMCP-gfp sequence from the phage-ubc-nls-ha-tdMCP-gfp construct (Addgene #40649) [37] was cloned into the pEGFP-C1 vector (Clontech). The pUBC-ha-tdMCP-GFP plasmid was generated by removing the NLS from the original vector. The pUBC-NLS-ha-tdMCP and pUBC-NLS-ha-tdMCP-Stau2 vectors were generated by extracting the UBC-NLS-ha-tdMCP sequence from the original vector and cloning the 62-kD isoform of mouse Stau2 in frame in the pEGFP-C1 vector (Clontech) in place of EGFP. The CMV-PSD95-tagRFPt vector was generated by cloning the PSD-95 ORF into the ptagRFPt-N1 vector (Robert H. Singer, USA). The pCMV-tagRFPt-Stau2 vector was generated by cloning the ORF of the 62-kD isoform of mouse Stau2 into the ptagRFPt-C1 vector (Robert H. Singer, USA). The pCMV-tdTomato vector was generated by cloning the ORF of tdTomato (Dieter Edbauer, Germany) into the ptagRFPt-C1 vector (Robert H. Singer, USA) in place of tagRFPt. The lentiviral packaging plasmids psPAX2 and pcDNA3.1-VSV-G have previously been described [30] . Lentiviral plasmids pFu3a-H1-sh-NTC-pCaMKIIα-tagRFP and pFu3a-H1-sh-Stau2-2-pCaMKIIα-tagRFP were generated by exchanging the UBC promoter for the CaMKIIα promoter from previously published FUW based vectors [30] . Lentivirus production Control sh-NTC and sh-Stau2-2 lentiviral particles were generated from HEK-293 cells cotransfected with the plasmids psPAX2, pcDNA3.1-VSV-G and either pFu3a-H1-sh-NTC-pCaMKIIα-tagRFP or pFu3a-H1-sh-Stau2-2-pCaMKIIα-tagRFP, respectively, using calcium phosphate coprecipitation. Supernatants were filtered (0.45 µm RVDF Millex-HV; Millipore), concentrated by ultracentrifugation (65,000 g , 140 min, SW 32 Ti rotor; Beckman Coulter) and resuspended in Opti-MEM™ (Life Technologies) [30] . Single molecule FISH Single molecule fluorescent in situ hybridization (smFISH) [40] was performed with slight modifications. Briefly, cells were fixed in 4% paraformaldehyde (PFA) for 20 min and permeabilized in 70% ethanol overnight at 4 °C, followed by two rounds of DNase treatment for 1 h each at 37 °C to remove plasmid DNA. Hybridization of ten unique Cy3-labelled antisense-MS2 probes was performed overnight at 37 °C. Coverslips were mounted using Prolong Gold antifade mounting medium (Invitrogen). The following set of ten Cy3 conjugated probes were used (5′–3′, X = aminoallyl-modified T): Probe 1 (nt 19–65): AXCGAGCGCATAAACCCXAATGGTGTTTACAAATGGXGGTAGTCCTACCXA; Probe 2 (nt 86–130): AXAAACGACCAGAGXGTATTTCTCTCTGATACGCXGCGTACTCGTCAXA; Probe 3 (nt 136–180): AXATTGTGCGGTCGCXGACTGATACTTCTAGXCATCCGTTTGTCTAGXA; Probe 4 (nt 186–231): AXGCTTGTAGTCAXAGCCTTAGCTTGGGTTATTACXCCAAGATCACCGXA; Probe 5 (nt 238–282): AXGGGTGGAAGCCTTACXGATGCTTCCGGTCCATXCTAATACTATGGXA; Probe 6 (nt 293–340): AXCCAGTAGTCTTGGACCCCXTGAATACTACTGTTATTCXAATCCGTCACXA; Probe 7 (nt 29–74): AXCCTAGTGGTACGCAGAXCATACCGTATTCGTGTAXGATTACATGGGXA; Probe 8 (nt 80–124): AXAATCATTCTAGTGAXATGATTCTGTGCCGCXACTGCTGGCACCGTXA; Probe 9 (nt 130–175): AXCGTCCTGATAGGCXGTACTCATGCCTACAACCXTCGATAATTCTGAXA; Probe 10 (nt 184–229): AXGTGTATTCATCTXAGCTGAGTGCTCTAAXGATGCACTACAGGACGCXA. Immunostaining For immunostaining [28] neurons were washed with warm Hanks′ Balanced Salt Solution (HBSS) and then fixed with warm 4% PFA in HBSS for 10 min. Fixed cells were washed with HBSS and permeabilized with 0.1% Triton X-100 in HBSS for 5 min. The following antibodies were used: (i) polyclonal antibodies, i.e. selfmade rabbit anti-Stau2 [53] , guinea pig anti-VGLUT1 (Synaptic Systems, 419005); (ii) secondary antibodies, i.e. donkey anti-rabbit and goat anti-guinea pig Alexa555 or Alexa647 conjugated (Life Technologies, A31572, A31573, A21450). Coverslips were mounted on slides with Prolong antifade mounting medium (Invitrogen). Chemical treatments To inhibit neuronal activity, cells were preincubated with 100 µM 6-cyano-7-nitroquinoxaline-2,3-dione (CNQX; Sigma, #C127), 50 µM 2-amino-5-phosphonopentanoic acid (AP5; Sigma, #A8054) and 1 µM tetrodotoxin (TTX; Abcam, #ab120055) in NMEM+B27 for 1 h at 37 °C. Media were exchanged for HBSS supplemented with 20 mM HEPES pH = 7.3, 100 µM CNQX, 50 µM AP5 and 1 µM TTX prior to imaging at the microscope. Vehicle treated cells were incubated with equivalent amount of DMSO. For cortical neurons, transfected cells were treated for 4 h with the aforementioned conditions and then lysed. RNA extraction, cDNA synthesis and qRT-PCR Total RNA was extracted with the RNeasy Mini Kit (Qiagen). cDNA was generated from 400 ng of total RNA, using Superscript III TM reverse transcriptase (Invitrogen) and 2.5-μM T20 primers according to the manufacturer’s instructions (+RT). As control for the presence of genomic DNA, equivalent reactions were made in the absence of reverse transcriptase (−RT). Quantitative real time PCR (qRT-PCR) was performed in duplicate from a 1:5 dilution of the stock cDNA, with a home-made SYBR Green Master Mix, with the LightCycler 96 System (Roche). The concentration of primers in the reaction was previously optimized to achieve 95–105% efficiency. Five microliters of an equimolar solution containing both forward and reverse primers were added to the reaction. Relative differences in RNA levels were calculated according to the 2 −ΔΔCt method [54] and normalized against either 18 S ribosomal RNA, peptidylprolyl isomerase A ( ppia ) mRNA or Kanamycin-resistance ( Km ) mRNA. The sequences of the primers were (5′–3′): 18S_f: GAAACTGCGAATGGCTCATTAAA; 18S_r: CCACAGTTATCCAAGTAGGAGAGGA; ppia_f: GTCAACCCCACCGTGTTCTT; ppia_r: CTGCTGTCTTTGGAACTTTG; KmR_f: TGCCTGCTTGCCGAATATCA; KmR_r: ATATCACGGGTAGCCAACGC; LacZ_f: CGCTGGATAACGACATTGGC; LacZ_r: TCGTAATCAGCACCGCATCA; Stau2_f: GAACATCTCCTGCTGCTGAAG; Stau2_r: ATCCTTGCTAAATATTCCAGTTGT. Microscopy Live-cell imaging was performed on a Zeiss Cell Observer spinning disk system consisting of a Zeiss Z1 Axio Observer microscope including a Plan-Apochromat 63x objective, a Yokogawa CSU-X1 spinning disk unit with 4 laser lines (405 nm 20 mW; 488 nm 50 mW, 561 nm 75 mW and 638 nm 75 mW) and an Evolve 512 Delta EMCCD Camera. For temperature control, a custom made EMBL environmental chamber (EMBLEM) was used. A 523/610 HC dual-band filter (AHF) was applied to reduce acquisition delay between channels during dual-color imaging. Hippocampal neurons were imaged at 36 °C in HBSS (Life Technologies) supplemented with 20 mM HEPES buffer pH 7.3 (Sigma Aldrich). Time-lapse images were acquired for the duration of 1, 3.5, or 10 min, with an approximate frame rate of ~15.3 fps for single channel acquisitions and ~4.7 fps for two-channel acquisitions with a 80 ms delay between channels. Cells were selected for proper expression of plasmids as well as for cell morphology and cell viability. Imaging of fixed cells was performed on a Zeiss Z1 Axio Observer microscope including a Plan-Apochromat 63x objective, a COLIBRI.2 LED or a HXP 120 C light source and the Axiocam 506 mono camera. Two-photon imaging and glutamate uncaging [55] , [56] were carried out by using a single laser (Mai Tai HP; Newport-Spectra Physics, Santa Clara, CA, USA), which was tuned to 930-nm excitation wavelength for 2-photon imaging and 720 nm for uncaging. In brief, recordings were performed at 35 °C in ACSF (in mM: 127 NaCl, 2.5 KCl, 25 NaHCO 3 , 1.25 NaH 2 PO 4 , 4 CaCl 2 , 25 d -glucose; in µM: 1 TTX, 10 D-serine; pH 7.4; saturated with carbogen) on a custom two-photon laser-scanning microscope (objective: 60×, 0.9 numerical aperture; Olympus, Tokyo, Japan). In some experiments, the ACSF contained 2 mM CaCl 2 , 1 mM MgCl 2 and no TTX and d -serine. Data obtained under these conditions were similar and pooled. MNI-caged l -glutamate was applied in the bath solution at 1.25 or 2.5 mM. Uncaging protocol: 30 pulses at 0.5 Hz, 4 ms pulse duration, wavelength 720 nm, 20 mW at the objective back aperture. At least six baseline image stacks (256 × 256 pixels, pixel size 0.105 or 0.125 µm) were recorded every 30 s on two channels (GFP, tdTomato) before glutamate uncaging was performed close to the dendritic spine to be stimulated. At 120 s or 150 s after stimulation, time-lapse imaging was resumed every 30 s until 5 min after stimulation, then every 60 s until 30 min and continued every 5 min until 60 min after stimulation. Image data analysis Time-series image data of reporter mRNAs was analyzed by kymographs. Dendritic 40-µm segments at ≥20 µm from the cell body were selected and straightened in ImageJ. The KymographTracker plugin of the ICY Bioimaging software [57] , [58] was used to generate kymographs and to trace and extract single tracks. Only movements longer than 1.5 µm were considered for analysis. Tracks were terminated when a particle stopped, changed direction or left the region of interest (ROI). Average speed and displacement were obtained by calculating the mean. Anterograde and retrograde tracks were counted to calculate the percent of anterograde transport. The sum of anterograde and retrograde displacement lengths was used to calculate the percent of total anterograde displacement. Dual-color kymographs were generated by overlaying identical regions of interest from two separate channels. Events in dual-color kymographs were manually selected and distances were manually measured in ImageJ (line tool), aided by a custom written ImageJ macro script (available upon request). 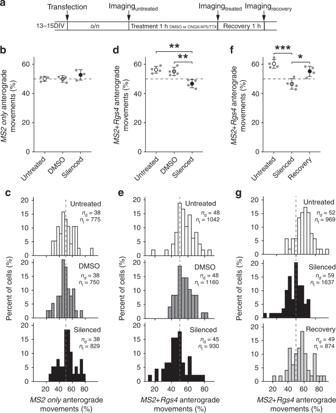Fig. 3 Inhibition of neuronal activity abolishesRgs43′-UTR-dependent transport bias.aScheme of experimental outline. Dot plots (b,d,f) and histograms (c,e,g) displaying percentage of anterograde movingMS2 only(b,c) orMS2+Rgs43′-UTR (d–g) reporter mRNA granules in rat hippocampal neurons, untreated, vehicle treated (DMSO) or silenced (100 µM CNQX, 50 µM AP5, 1 µM TTX) and after 1-h recovery. Data represent mean ± standard deviation of 3–4 independent experiments (individual experiments shown as gray dots). Asterisks representp-values assessed by Tukey’s test post-hoc to one-way ANOVA analysis (*p< 0.05, **p< 0.01, ***p< 0.001). Data were obtained from 40-µm dendritic segments at a minimal distance of 20 µm from the cell body. At least 10 dendrites/condition/experiment were analyzed. Total number of dendrites (nd) and tracks (nt) analyzed per condition are indicated. Only displacements ≥1.5 µm were considered for analysis Data were processed and subjected to statistical analyses in R [59] . RNA signal intensity of PSD-95 labelled postsynaptic densities was analyzed within the synaptic masks generated by the xsParticle Tracker ImageJ plugin [60] , [61] .Time series of the measured, background corrected reporter RNA signal was fitted with a series of constants using the rpart package of R [62] . Minimum duration of a single constant fit was set to five frames (~1 s). The 5th percentile of the RNA signal intensity distribution measured in every 100 frames (for correction of photobleaching, Supplementary Fig. 6e, f ) was used as the signal corresponding to a single reporter RNA molecule. Changes between two adjacent fitted constants, whose absolute value exceeded this threshold were quantified as docking and undocking events, depending on the sign of the change. For deconvolution, z-stacks with 25 images at an interval of 0.26 µm were acquired, covering a total distance of 6.24 µm. Z-stacks were subjected to deconvolution using the constrained iterative quantitative restoration method of the Zeiss ZEN software deconvolution module. For analysis of time-lapse series with glutamate uncaging, individual frames from image stacks were median filtered (5 × 5 pixel window) and maximum intensity projections generated. Dendritic spine size (tdTomato fluorescence) was determined as integrated fluorescence within a ROI containing the spine and subtracting integrated background signal from a ROI of the same size placed outside of any structure. To control for stimulus specific changes in spine size, the size of neighboring unstimulated spines or of an adjacent dendritic region was determined in the same way. Data were analyzed with custom routines written in MATLAB (version R2018b, MathWorks, Natick, MA, USA). 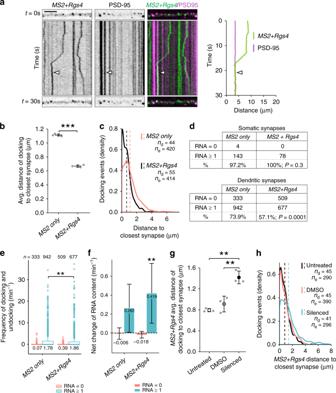Fig. 4 Rgs43′-UTR mediates mRNA recruitment to synapses dependent on neuronal activity.aRepresentative dual-color kymograph showingMS2+Rgs43′-UTR reporter mRNA (green) and PSD-95-tagRFPt (magenta) from a dendrite of a rat hippocampal neuron. First and last frames are shown at top and bottom. Scale bar 5 µm. Extracted track (right) of an mRNA granule docking at a PSD-95 positive area indicated by arrowheads. Distance ofMS2 onlyorMS2+Rgs43′-UTR reporter mRNA docking events to closest PSD-95 positive cluster in neurons displayed as dot plot (b) and density plot (c).dDistribution ofMS2 onlyorMS2+Rgs4reporter mRNA-positive (estimated RNA number ≥1 att= 0 s) and -negative (RNA = 0 att= 0 s) PSD-95-tagRFPt clusters in soma and dendrites.P-valuesof Chi2tests against control are indicated.eIntegrated frequency of reporter docking and undocking events at dendritic synapses. Number of observations and population means are indicated.fAverage net change ofMS2 onlyorMS2+Rgs4mRNA content at mRNA reporter-positive or -negative synapses per min, calculated from estimated reporter molecules docking or undocking at synapses per event. Numbers indicate mean value of net RNA level change. Error bars represent 95% confidence intervals. ** indicates significant (α= 0.01) difference compared to zero (null hypothesis, two sided one-samplet-test). Distance ofMS2+Rgs43′-UTR reporter mRNA docking events to closest PSD-95 positive cluster under untreated, vehicle treated (DMSO) or silenced (100 µM CNQX, 50 µM AP5, 1 µM TTX) conditions displayed as dot plot (g) and density plot (h). Data represent mean ± standard deviation of three independent experiments (individual experiments shown as gray dots;b,g). Dashed lines represent mean values of single data points (c,h). Asterisks representp-values obtained by Student’sttest (b), Mann WhitneyUtest (e) or Tukey’s test post-hoc to one-way ANOVA analysis (g) (**p< 0.01, ***p< 0.001). Data were obtained from 40-µm dendritic segments at a minimal distance of 20 µm from the cell body. At least 10 dendrites/condition/experiment (a–c,g,h) or 12 neurons/condition (d–f) from 3 independent biological replicates were analyzed. Total number of dendrites (nd), events (ne) and synapses (n) analyzed per condition are indicated mRNA granules were manually quantified in a 5-µm dendritic radius centered at the stimulated spine. To compensate for fluctuations due to ongoing transport two time points before (~7–4 and ~2 min) and after (40 and 45 min) uncaging were averaged respectively. Statistical analysis R software or DeltaGraph Prism v8.0 were used for all data processing, plotting and statistical analysis [59] , [63] , [64] , [65] . Figures represent mean ± standard deviation of at least three independent biological replicates, unless otherwise stated. Asterisks represent p -values obtained by either Student’s t test, Tukey’s test post-hoc to one-way ANOVA analysis using the average values per experiment or pairwise Mann–Whitney U tests (* p < 0.05, ** p < 0.01, *** p < 0.001), as indicated. The F -value evaluates whether the variance between the means of populations is significantly different (Fisher–Snedecor’s F distribution). The degrees of freedom are indicated as subscript. Significant levels ( α ) are provided for Fig. 4f and Supplementary Fig. 4i . 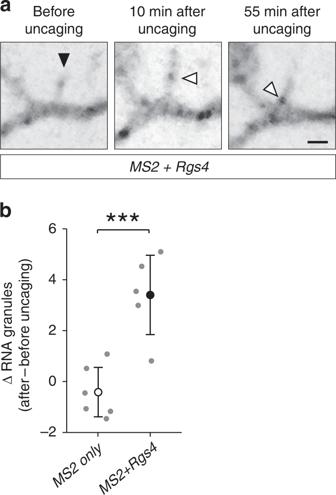Fig. 5 Local glutamate uncaging at spines triggersRgs43′-UTR-dependent mRNA recruitment.aRepresentative GFP fluorescence of a hippocampal neuron cotransfected with theMS2+Rgs43′-UTR reporter and tdMCP-GFP constructs before (left panel) and after (middle, right panels) local glutamate uncaging. Black arrowhead denotes the uncaging spot at dendritic spine. White arrowheads indicate GFP positiveMS2+Rgs4reporter mRNA granules. Scale bar 2 µm.bDot plot displaying the change in RNA granule number 40–45 min after uncaging compared to before uncaging within 5 µm of the stimulated spine. Data represent mean ± standard deviation (individual neurons shown as gray dots). Asterisks representp-values obtained by Student’sttest (***p< 0.001). Data were obtained from six dendrites forMS2 only(five neurons of four biological replicates) and five dendrites forMS2+Rgs4reporter mRNAs (five neurons of five biological replicates), respectively 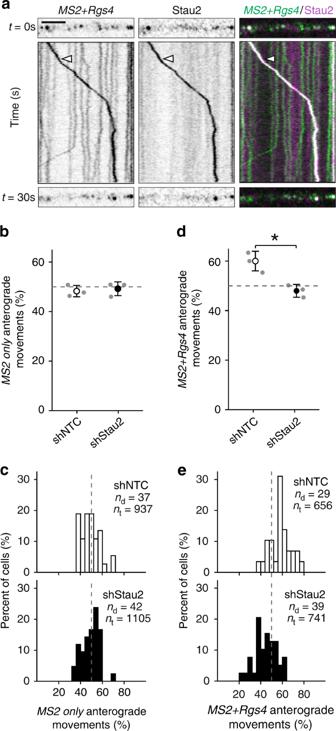Fig. 6 Stau2 regulatesRgs43′-UTR-dependent transport.aRepresentative dual-color kymograph showingMS2+Rgs43′-UTR reporter mRNA (green) and tagRFPt-tagged Stau2 (magenta) from a dendrite of a rat hippocampal neuron. First and last frames are shown at top and bottom. Arrowheads indicate anMS2+Rgs4reporter and Stau2 positive RNA granule undergoing cotransport. Scale bar 5 µm. Dot plots (b,d) and histograms (c,e) displaying percentage of anterograde movingMS2 onlyorMS2+Rgs43′-UTR reporter mRNA granules in shNTC and shStau2 transduced hippocampal neurons. NTC non-targeting control. Data represent mean ± standard deviation of three independent experiments (individual experiments shown as gray dots). Asterisks representp-values obtained by Student’sttest (*p< 0.05). Data were obtained from 40-µm dendritic segments at a minimal distance of 20 µm from the cell body. Total number of dendrites (nd) and tracks (nt) analyzed per condition are indicated. Only displacements ≥1.5 µm were considered for analysis Reporting summary Further information on research design is available in the Nature Research Reporting Summary linked to this article.